Single-cell dynamics of the chromosome replication and cell division cycles in mycobacteria During the bacterial cell cycle, chromosome replication and cell division must be coordinated with overall cell growth in order to maintain the correct ploidy and cell size. The spatial and temporal coordination of these processes in mycobacteria is not understood. Here we use microfluidics and time-lapse fluorescence microscopy to measure the dynamics of cell growth, division and chromosome replication in single cells of Mycobacterium smegmatis . We find that single-cell growth is size-dependent (large cells grow faster than small cells), which implicates a size-control mechanism in cell-size homoeostasis. Asymmetric division of mother cells gives rise to unequally sized sibling cells that grow at different velocities but show no differential sensitivity to antibiotics. Individual cells are restricted to one round of chromosome replication per cell division cycle, although replication usually initiates in the mother cell before cytokinesis and terminates in the daughter cells after cytokinesis. These studies reveal important differences between cell cycle organization in mycobacteria compared with better-studied model organisms. The bacterial cell cycle comprises interlocking cycles of chromosome replication and segregation as well as cell division and separation. These periodic events must be coordinated in space and time to maintain chromosomal integrity and balanced cell growth. The mechanisms that link the chromosome replication cycle to the cell division cycle have been the subject of intensive investigation for many years. However, the current state of knowledge is largely based on studies in a small number of fast-growing model organisms, especially Escherichia coli , Bacillus subtilis and Caulobacter crescentus . Comparisons between these organisms make it clear that cell cycle regulation differs between them in some fundamental aspects. For example, E. coli and B. subtilis exhibit multifork chromosome replication during rapid growth under nutrient-rich conditions, whereas C. crescentus does not reinitiate chromosome replication until the previous round of replication as well as cell division have been completed [1] , [2] . It is not known how events of the chromosome replication and cell division cycles are coordinated in the distantly related and more slowly growing microorganisms of the genus Mycobacterium . In exponentially growing cell populations, the discontinuous processes of chromosome replication/segregation and cell division/separation must also be coordinated with the continuous increase in cell biomass in order to maintain a constant cell-size distribution. A long-standing debate in the field of cell biology concerns the question whether growth of single cells follows a linear or exponential pattern [3] , [4] . Linear growth implies that the speed of growth remains constant between birth and division and does not scale with cell size. Exponential growth implies that the speed of growth accelerates in proportion to increasing cell size. In practice, distinguishing between linear and exponential patterns of single-cell growth is technically challenging because the respective growth curves exhibit similar shapes, and highly precise measurements are required to distinguish between them [3] , [5] , [6] . Recent studies using a variety of experimental techniques lend support to the hypothesis that growth of single cells is size-dependent and approximately exponential in E. coli , B. subtilis , budding yeast and mammalian cells [5] , [6] , [7] . Most rod-shaped bacteria, including E. coli and B. subtilis , grow by inserting new cell-wall material into their lateral sidewalls [8] . Consequently, the surface area that is available for insertion of new cell-wall material increases continuously from birth to next division. In contrast, rod-shaped Actinobacteria, including organisms in the genus Mycobacterium , grow by inserting new cell-wall material exclusively at the cell poles [9] , [10] , [11] , [12] , [13] . As these cells grow by extending their length while maintaining an approximately constant width, the surface area available for insertion of new cell-wall material at the cell poles does not change appreciably between birth and division. These contrasting modes of cell growth suggest that the pattern of single-cell growth might differ between bacteria that grow by sidewall extension (exponential growth) versus bacteria that grow by tip extension (linear growth) [14] . It has also been proposed that cell division might not be coupled to cell size in bacteria that grow by tip extension, which do not have to pause growth in order to build a new division septum [14] . To the best of our knowledge, these hypotheses have not been addressed experimentally. Recently, it was reported that Mycobacterium smegmatis grows in an unusual unipolar manner by preferential extension of the old cell pole, whereas the new cell pole remains quiescent until the next cell division has been completed [12] , [15] , [16] . Unipolar growth was hypothesized to give rise to asymmetric cell division, resulting in sibling cells of unequal sizes and growth velocities, with larger old-pole cells growing faster than their smaller new-pole siblings [15] . As a possible consequence of differences in their growth velocities, old-pole cells were reported to be more susceptible to killing by antibiotics than new-pole cells [15] . In this study, we investigate the dynamics of chromosome replication, cell growth and cell division in single cells of M. smegmatis using fluorescent reporter strains, microfluidic culture systems and time-lapse microscopy. We show that growth of single cells is size-dependent and bipolar, with old and new poles elongating at equal velocities following separation of sibling cells. Moreover, old-pole and new-pole sibling cells differ in birth length and elongation velocity (absolute length increase over time, μm h −1 ) but not in elongation rate (relative length increase over time, h −1 ) or antibiotic sensitivity. Although multifork chromosome replication apparently does not occur in M. smegmatis , organization of the cell cycle is unusual inasmuch as chromosome replication can initiate before or after the previous round of cell division has been completed. Cytokinesis coincides with Wag31 localization to the septum We measure cell division cycle dynamics in single cells of M. smegmatis by growing the cells in a microfluidic device and imaging them by time-lapse fluorescence microscopy [17] . Cell division events are visualized using a merodiploid reporter strain expressing a Wag31-GFP (green-fluorescent protein) fusion protein ( Supplementary Movie 1 , Supplementary Table S1 ). Wag31 is an essential late-division protein that localizes to the division septum and remains associated with the newly formed cell poles after physical separation of sibling cells [11] , [18] , [19] . Growth of the Wag31-GFP strain in the presence of the membrane-staining fluorescent dye FM4-64 allows visualization of the early stages of septum biogenesis ( Fig. 1a and Supplementary Movie 2 ). Analysis of time-lapse image series confirms that the septum in mycobacteria is not always placed exactly at midcell [12] , [15] , [16] . In the majority of cells, septum position is skewed towards the new pole ( Fig. 1b and Supplementary Fig. S1a ). Asymmetric positioning of the septum is independent of cell length ( Supplementary Fig. S1b ). 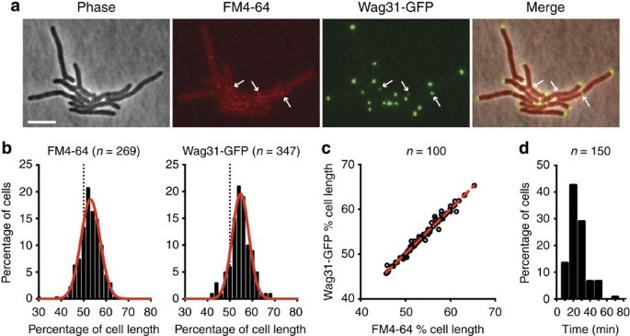Figure 1: Single-cell dynamics of septum formation. (a–d) Time-lapse microscopy of bacteria expressing Wag31-GFP and stained with the fluorescent membrane dye FM4-64. Images recorded at 10-min intervals. This experiment was repeated two times with similar results. (a) Phase-contrast and fluorescence images. Arrows indicate colocalization of Wag31-GFP with FM4-64-stained septa. Scale bar, 3 μm. (b) Frequency distributions of the positions of septal FM4-64 (n=269) and Wag31-GFP (n=347) as a percentage of cell length. Red line, data fitted by a Gaussian function. Vertical dotted line, midcell. Septum placement is skewed towards the new pole at 54±5% (FM4-64) or 55±4% (Wag31-GFP) of total cell length (percent values are mean±s.d.). (c) Positions of septal FM4-64 and Wag31-GFP in single cells as a percentage of cell length (n=100). Red line, data fitted by a linear function. (d) Frequency distribution of the time interval between septum initiation (appearance of FM4-64-stained membrane invagination) and localization of Wag31-GFP to the septum (n=150). Figure 1: Single-cell dynamics of septum formation. ( a – d ) Time-lapse microscopy of bacteria expressing Wag31-GFP and stained with the fluorescent membrane dye FM4-64. Images recorded at 10-min intervals. This experiment was repeated two times with similar results. ( a ) Phase-contrast and fluorescence images. Arrows indicate colocalization of Wag31-GFP with FM4-64-stained septa. Scale bar, 3 μm. ( b ) Frequency distributions of the positions of septal FM4-64 ( n =269) and Wag31-GFP ( n =347) as a percentage of cell length. Red line, data fitted by a Gaussian function. Vertical dotted line, midcell. Septum placement is skewed towards the new pole at 54±5% (FM4-64) or 55±4% (Wag31-GFP) of total cell length (percent values are mean±s.d.). ( c ) Positions of septal FM4-64 and Wag31-GFP in single cells as a percentage of cell length ( n =100). Red line, data fitted by a linear function. ( d ) Frequency distribution of the time interval between septum initiation (appearance of FM4-64-stained membrane invagination) and localization of Wag31-GFP to the septum ( n =150). Full size image In single cells, Wag31-GFP colocalizes with the FM4-64-stained septum ( Fig. 1c ), and the timing of Wag31-GFP localization to the septum is consistent with that of a late-division protein. Initiation of septation is visible as an invagination of the FM4-64-stained membrane at midcell, which precedes Wag31-GFP septal localization by 25±11 min (mean±s.d.) ( Fig. 1d ). These observations suggest that localization of Wag31 to the cell division septum might coincide with closure of the septum, resulting in cytoplasmic compartmentalization (cytokinesis) of the newly born sibling cells. In this study, the time of cytokinesis is defined as the time when sibling cells become compartmentalized such that diffusive mixing between their cytosolic components no longer occurs. Fluorescence loss in photobleaching (FLiP) assays [20] , [21] can be used to determine the timing of cytoplasmic compartmentalization relative to Wag31 septal localization in single cells ( Fig. 2a ). For this purpose, we use a reporter strain expressing Wag31-GFP to mark the cell division septum and a red-fluorescent protein (DsRed2) as a freely diffusing cytosolic marker. In time-lapse experiments we find that a septal Wag31-GFP signal of 7 a.u. is the minimum signal detectable by visual inspection of images ( Fig. 2b ). In cells with a septal Wag31-GFP signal <7 a.u., DsRed2 is equally bleached in the cell ends proximal and distal to the laser focus, indicating that compartmentalization of the mother cell cytoplasm has not yet occurred ( Fig. 2c ). In contrast, in cells with a septal Wag31-GFP signal >7 a.u. we observe minimal bleaching of DsRed2 in the cell ends distal to the laser focus, similar to bleaching of control bystander cells, indicating that cytokinesis of the daughter cells is complete ( Fig. 2c ). FLiP experiments with FM4-64 membrane staining and genetically expressed GFP as a freely diffusing cytosolic marker ( Supplementary Fig. S1c and Supplementary Fig. S1e ) reveal that cytokinesis is completed within 20–30 min of septum initiation ( Supplementary Fig. S1d ). This timing is similar to the interval of time between septum initiation (appearance of septal FM4-64 staining) and septal localization of Wag31-GFP ( Fig. 1d ). Even at late stages of septal biogenesis, before and after cytokinesis, the septum is not visible in phase-contrast images. 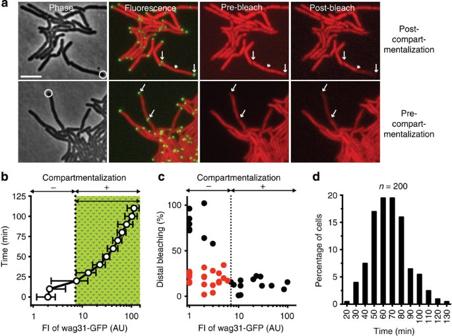Figure 2: Cytokinesis coincides with the localization of Wag31-GFP to the septum. (a–d) Time-lapse microscopy of bacteria expressing Wag31-GFP and cytosolic DsRed. Images recorded at 10-min intervals. (a) Representative FLiP experiments showing examples of a mother cell precompartmentalization (lower panels) and two sibling cells post compartmentalization (upper panels). Phase-contrast and fluorescence images recorded before and after photobleaching with a laser pulse. White circles (‘Phase’ panels) indicate foci of the bleaching laser. ‘Fluorescence’ panels represent GFP and DsRed channels. ‘Pre-bleach’ and ‘Post-bleach’ panels represent DsRed channel. Arrows, polar localization of Wag31-GFP. Arrowheads (upper panels), septal localization of Wag31-GFP. Scale bar, 3 μm. (b) Time-dependent increase in septal Wag31-GFP fluorescence intensity (FIWag31-GFP) in arbitrary units (n=25). Green shading indicates that sibling cells are compartmentalized. (c) Percent decrease in fluorescence intensity in the distal end of the cell versus FIWag31-GFPin arbitrary units (n=25). Black symbols, bleached cells. Red symbols, control cells adjacent to bleached cells. Vertical dotted line, value of FIWag31-GFPcorresponding to cytoplasmic compartmentalization (cytokinesis) of sibling cells. (d) Frequency distribution of the time interval between cytokinesis and physical separation of sibling cells (n=200). This experiment was repeated three times with similar results. Figure 2: Cytokinesis coincides with the localization of Wag31-GFP to the septum. ( a – d ) Time-lapse microscopy of bacteria expressing Wag31-GFP and cytosolic DsRed. Images recorded at 10-min intervals. ( a ) Representative FLiP experiments showing examples of a mother cell precompartmentalization (lower panels) and two sibling cells post compartmentalization (upper panels). Phase-contrast and fluorescence images recorded before and after photobleaching with a laser pulse. White circles (‘Phase’ panels) indicate foci of the bleaching laser. ‘Fluorescence’ panels represent GFP and DsRed channels. ‘Pre-bleach’ and ‘Post-bleach’ panels represent DsRed channel. Arrows, polar localization of Wag31-GFP. Arrowheads (upper panels), septal localization of Wag31-GFP. Scale bar, 3 μm. ( b ) Time-dependent increase in septal Wag31-GFP fluorescence intensity (FI Wag31-GFP ) in arbitrary units ( n =25). Green shading indicates that sibling cells are compartmentalized. ( c ) Percent decrease in fluorescence intensity in the distal end of the cell versus FI Wag31-GFP in arbitrary units ( n =25). Black symbols, bleached cells. Red symbols, control cells adjacent to bleached cells. Vertical dotted line, value of FI Wag31-GFP corresponding to cytoplasmic compartmentalization (cytokinesis) of sibling cells. ( d ) Frequency distribution of the time interval between cytokinesis and physical separation of sibling cells ( n =200). This experiment was repeated three times with similar results. Full size image We conclude that these two events—cytokinesis and localization of Wag31-GFP to the septum—occur very close together in time. Thus, in time-lapse series we can define the interdivision time of single cells as the time interval between two consecutive Wag31-GFP septal-localization events ( Supplementary Fig. S1f ). Time-lapse analysis also revealed that there is a variable and substantial time interval of 67±20 min (mean±s.d.) between cytokinesis and sibling cell separation resulting in the formation of new cell poles ( Fig. 2d ). These points are critical to interpreting the growth patterns of single cells, as discussed in the following section. Single cells elongate in a bipolar manner Recently, it was reported that single cells of M. smegmatis elongate in an unusual unipolar manner [15] . According to the proposed model, which is reproduced in Fig. 3a , between birth and next division the new cell pole is quiescent and elongation occurs exclusively at the old cell pole. Here, we re-examine this issue by pulse labelling the cell wall with green-fluorescent amine-reactive dye and measuring the extension of the unlabelled poles over time ( Supplementary Fig. S2a ), as described [15] . In these experiments, we use a reporter strain expressing a Wag31-mCherry fusion protein to monitor cytokinesis (see above) and phase imaging to monitor cell separation ( Supplementary Movie 3 ). 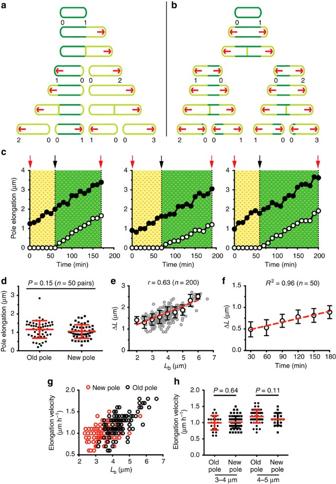Figure 3: Growth of single cells is bipolar and size-dependent. (a) Schematic of unipolar cell growth reproduced from Aldridgeet al15. A surface-labeled cell (dark green) elongates exclusively from one pole (red arrow). Division generates sibling cells that elongate exclusively from old poles, whereas new poles do not elongate until the next cell division cycle. Numbers indicate pole ages. (b) Schematic of bipolar cell growth based on data presented in this paper. A surface-labeled cell (dark green) grows from both poles (red arrows). Cytokinesis and separation generate sibling cells that elongate at equal velocities from both poles (red arrows). Numbers indicate pole ages. (c–h) Time-lapse microscopy of bacteria expressing Wag31-GFP. Images recorded at 10-min intervals. (c) Three representative single-cell time traces showing elongation of the old pole (black circles) and new pole (white circles) during one cell division cycle. Red arrows indicate successive cytokinesis events marked by the localization of Wag31-GFP to the septum. Black arrows indicate physical separation of sibling cells. Yellow shading indicates period between cytokinesis and sibling cell separation. Green shading indicates period between sibling cell separation and next cytokinesis. (d) Elongation of old and new cell poles during the period of bipolar growth between sibling cell separation and next cytokinesis. Mann–Whitney rank sum test,P=0.15 (n=50). (e) Incremental increase in cell length (ΔL) during the first 90 min after birth versus length of the cell at birth (Lb). Grey circles, ΔLof single cells. Black circles, mean ΔL±s.d. for cells binned byLb. Dashed red line, data fitted to a linear function. Pearson's correlation coefficient,r=0.63 (n=200). (f) Mean ΔL±s.d. binned in 30-min time intervals starting from birth (0 min). Dashed red line, data fitted to a linear function. Coefficient of determination,R2=0.96 (n=50). (g) Elongation velocity (μm h−1) versus length at birth (Lb) for new-pole cells (red circles,n=100) and old-pole cells (black circles,n=100). (h) Elongation velocity (μm h−1) of new-pole cells and old-pole cells binned according to length at birth (Lb) in the rangesLb=3–4 μm (Student's unpairedt-test,P=0.64,n=23 for old-pole cells andn=61 for new-pole cells) andLb=4–5 μm (Student's unpairedt-test,P=0.11,n=56 for old-pole cells andn=19 for new-pole cells). Figure 3: Growth of single cells is bipolar and size-dependent. ( a ) Schematic of unipolar cell growth reproduced from Aldridge et al [15] . A surface-labeled cell (dark green) elongates exclusively from one pole (red arrow). Division generates sibling cells that elongate exclusively from old poles, whereas new poles do not elongate until the next cell division cycle. Numbers indicate pole ages. ( b ) Schematic of bipolar cell growth based on data presented in this paper. A surface-labeled cell (dark green) grows from both poles (red arrows). Cytokinesis and separation generate sibling cells that elongate at equal velocities from both poles (red arrows). Numbers indicate pole ages. ( c – h ) Time-lapse microscopy of bacteria expressing Wag31-GFP. Images recorded at 10-min intervals. ( c ) Three representative single-cell time traces showing elongation of the old pole (black circles) and new pole (white circles) during one cell division cycle. Red arrows indicate successive cytokinesis events marked by the localization of Wag31-GFP to the septum. Black arrows indicate physical separation of sibling cells. Yellow shading indicates period between cytokinesis and sibling cell separation. Green shading indicates period between sibling cell separation and next cytokinesis. ( d ) Elongation of old and new cell poles during the period of bipolar growth between sibling cell separation and next cytokinesis. Mann–Whitney rank sum test, P =0.15 ( n =50). ( e ) Incremental increase in cell length (Δ L ) during the first 90 min after birth versus length of the cell at birth ( L b ). Grey circles, Δ L of single cells. Black circles, mean Δ L ±s.d. for cells binned by L b . Dashed red line, data fitted to a linear function. Pearson's correlation coefficient, r =0.63 ( n =200). ( f ) Mean Δ L ±s.d. binned in 30-min time intervals starting from birth (0 min). Dashed red line, data fitted to a linear function. Coefficient of determination, R 2 =0.96 ( n =50). ( g ) Elongation velocity (μm h −1 ) versus length at birth ( L b ) for new-pole cells (red circles, n =100) and old-pole cells (black circles, n =100). ( h ) Elongation velocity (μm h −1 ) of new-pole cells and old-pole cells binned according to length at birth ( L b ) in the ranges L b =3–4 μm (Student's unpaired t -test, P =0.64, n =23 for old-pole cells and n =61 for new-pole cells) and L b =4–5 μm (Student's unpaired t -test, P =0.11, n =56 for old-pole cells and n =19 for new-pole cells). Full size image During the period between cytokinesis and separation of newly born sibling cells ( Fig. 2d ), the new cell poles have not yet formed and growth occurs exclusively at the old cell poles (yellow shading in Fig. 3c ). In time-lapse series, separation of sibling cells is followed by a time interval (green shading in Fig. 3c ) during which both poles, new and old, elongate to the same extent ( Fig. 3d ). Our measurements of the elongation of isolated single cells ( Supplementary Movies 3 and 4 ) also reveal no significant difference in the elongation of the two cell poles ( Supplementary Fig. S2b,c ). These observations suggest an alternative model of the mycobacterial cell division cycle in which the old and new poles of individual cells elongate at equal velocities following a period of variable duration between cytokinesis and sibling cell separation ( Fig. 3b ). Elongation velocity of single cells is size-dependent Time-lapse microscopic analysis of M. smegmatis reveals a strong positive correlation between cell length at birth ( L b ) and incremental length (Δ L ) during the next 90 min after birth ( Fig. 3e ). Similarly, by measuring Δ L of single cells at 30-min intervals between birth and next division we find that as cells increase their length they elongate more rapidly ( Fig. 3f ). The overlap in frequency distributions of L b for new-pole and old-pole cells ( Fig. 3g ) permits comparison of the elongation velocities of cells with similar birth lengths in the range of 3–4 or 4–5 μm. These comparisons reveal that new-pole and old-pole cells that are similar in size also elongate at similar velocities ( Fig. 3h ). We conclude that old-pole cells tend to grow faster than their new-pole siblings not because of the difference in pole age per se but because old-pole cells tend to be larger at birth and elongation velocity is size-dependent. Sibling cells are equally sensitive to antibiotics Consistent with the observed patterns of asymmetric division and size-dependent growth of single cells, old-pole- and new-pole cells differ in their birth lengths ( Fig. 4a ), division lengths ( Supplementary Fig. S3a ) and elongation velocities ( Fig. 4b ) but not in their elongation rates ( Fig. 4c ) or interdivision times ( Supplementary Fig. S3b ). On average, old-pole siblings elongate more before dividing but without doubling their size, whereas new-pole siblings elongate less but double their size before dividing ( Supplementary Fig. S3c,d ). By tracking individual cell lineages through successive divisions, beginning with newborn cells with pole ages ‘0’ and ‘1’ ( Fig. 3b ), we find that L b increases from generations 0–1 to 0–3 before stabilizing ( Supplementary Fig. S4a ). Consistent with size-dependent growth of single cells, elongation velocity also increases from generations 0–1 to 0–3 before stabilizing ( Supplementary Fig. S4b ), whereas elongation rate ( Supplementary Fig. S4c ) and interdivision time ( Supplementary Fig. S4d ) remain constant. 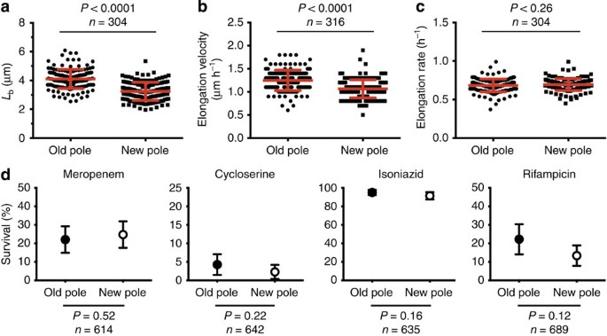Figure 4: Sibling cells do not differ in elongation rate or antibiotic sensitivity. (a–c) Time-lapse microscopy of bacteria expressing Wag31-GFP. Images recorded at 10-min intervals. Red lines and error bars indicate mean values±s.d.P-values, Student's unpairedt-test. This experiment was repeated three times with similar results. (a)Lb, length at birth of sibling cell pairs (P<0.0001,n=304). (b) Elongation velocity of sibling cell pairs (P<0.0001,n=316). (c) Elongation rate of sibling cell pairs (P=0.26,n=304). (d) Time-lapse microscopy of bacteria expressing Wag31-GFP. Images recorded at 10-min intervals. Percent survival of old-pole- and new-pole cells exposed for 8 h to twofold the MIC (minimum inhibitory concentration) of meropenem, cycloserine or rifampicin, or 10-fold the MIC of isoniazid. Percent survival indicates the fraction of regrowing cells after removal of antibiotic from the flow medium.P-values, Mann–Whitney rank sum test. Data are mean values±s.d. This experiment was repeated two times with similar results. Figure 4: Sibling cells do not differ in elongation rate or antibiotic sensitivity. ( a – c ) Time-lapse microscopy of bacteria expressing Wag31-GFP. Images recorded at 10-min intervals. Red lines and error bars indicate mean values±s.d. P -values, Student's unpaired t -test. This experiment was repeated three times with similar results. ( a ) L b , length at birth of sibling cell pairs ( P <0.0001, n =304). ( b ) Elongation velocity of sibling cell pairs ( P <0.0001, n =316). ( c ) Elongation rate of sibling cell pairs ( P =0.26, n =304). ( d ) Time-lapse microscopy of bacteria expressing Wag31-GFP. Images recorded at 10-min intervals. Percent survival of old-pole- and new-pole cells exposed for 8 h to twofold the MIC (minimum inhibitory concentration) of meropenem, cycloserine or rifampicin, or 10-fold the MIC of isoniazid. Percent survival indicates the fraction of regrowing cells after removal of antibiotic from the flow medium. P -values, Mann–Whitney rank sum test. Data are mean values±s.d. This experiment was repeated two times with similar results. Full size image The observation that asymmetric division yields sibling cells with different elongation velocities suggests that old-pole- and new-pole cells might display differential sensitivity to antibiotics. Consistent with this hypothesis, it has been reported that old-pole cells are more sensitive than new-pole cells to killing by meropenem, cycloserine and isoniazid, which target cell-wall biogenesis, whereas the opposite is true for rifampicin, which targets RNA polymerase [15] . In contrast, we find that there is no significant difference between old-pole- and new-pole cells with respect to killing by any of these antibiotics ( Fig. 4d ). We conclude that differences in the birth sizes and elongation velocities of old-pole and new-pole sibling cells do not result in differential sensitivity to killing by antibiotics under the experimental conditions used in our study. Non-canonical organization of the mycobacterial cell cycle The observed variation in single-cell elongation rates and interdivision times prompted us to investigate the relationship between the chromosome replication and cell division cycles in M. smegmatis . The timing and duration of the C period can be measured in single cells by using a dual fluorescent reporter strain that expresses Wag31-GFP to mark the cell division septum and a mCherry-DnaN fusion protein to mark the sliding processivity clamp of the DNA replisome complex [22] , [23] , [24] . In the cytoplasm of the dual reporter strain, appearance and disappearance of diffraction-limited mCherry-DnaN foci correspond to assembly and disassembly of the DNA replisome complex, respectively ( Fig. 5a and Supplementary Movie 5 ). In our experiments, we define the C period as the time interval between appearance and disappearance of mCherry-DnaN foci. At present, however, we cannot rule out the possibility that there might be a lag between replisome assembly and replication initiation or a lag between replication termination and replisome disassembly. 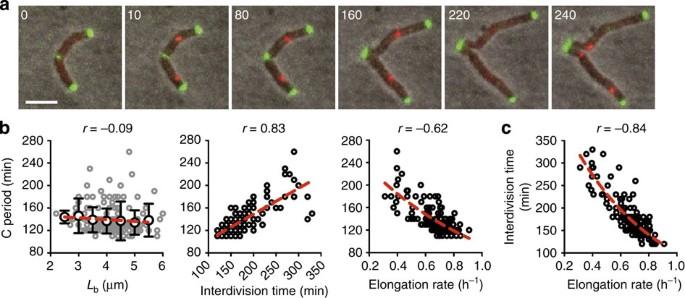Figure 5: Non-canonical organization of the chromosome replication and cell division cycles. (a–c) Time-lapse microscopy of bacteria expressing Wag31-GFP and mCherry-DnaN. Images recorded at 10-min intervals. This experiment was repeated three times with similar results. (a) Representative phase-contrast and fluorescence images recorded at the indicated time points (min). Scale bar, 3 μm. Green, Wag31-GFP. Red, mCherry-DnaN. (b) Duration of the C period versus birth length (Lb) (r=−0.09), interdivision time (r=0.83) and elongation rate (r=−0.62) of single cells. In theLbplot, grey circles represent the C period for single cells and black circles with error bars represent the mean C period duration±s.d. for cells binned byLb. Dashed red line, data fitted to a linear function.rvalues, Pearson's correlation coefficient (n=150). (c) Interdivision time versus elongation rate of single cells. Dashed red line, data fitted to a linear function. Pearson's correlation coefficient,r=−0.84 (n=150). Figure 5: Non-canonical organization of the chromosome replication and cell division cycles. ( a – c ) Time-lapse microscopy of bacteria expressing Wag31-GFP and mCherry-DnaN. Images recorded at 10-min intervals. This experiment was repeated three times with similar results. ( a ) Representative phase-contrast and fluorescence images recorded at the indicated time points (min). Scale bar, 3 μm. Green, Wag31-GFP. Red, mCherry-DnaN. ( b ) Duration of the C period versus birth length ( L b ) ( r =−0.09), interdivision time ( r =0.83) and elongation rate ( r =−0.62) of single cells. In the L b plot, grey circles represent the C period for single cells and black circles with error bars represent the mean C period duration±s.d. for cells binned by L b . Dashed red line, data fitted to a linear function. r values, Pearson's correlation coefficient ( n =150). ( c ) Interdivision time versus elongation rate of single cells. Dashed red line, data fitted to a linear function. Pearson's correlation coefficient, r =−0.84 ( n =150). Full size image Pedigree analysis reveals the organization of the chromosome replication and cell division cycles within a single-cell lineage derived from a common progenitor cell (for example, Supplementary Fig. S5 ). In our experiments, duration of the C period is 140±27 min (mean±s.d.) ( Supplementary Fig. S6a ) compared with an interdivision time of 180±45 min (mean±s.d.) ( Supplementary Fig. S6b and Supplementary Table S1 ). Although duration of the C period does not correlate with birth length, it does correlate with interdivision times and elongation rates of single cells ( Fig. 5b ). To a lesser extent, single-cell interdivision times and elongation rates also correlate with duration of the B period between division and initiation of DNA replication ( Supplementary Fig. S6c ) and the D period between the completion of DNA replication and division ( Supplementary Fig. S6d ). As the interdivision times of single cells increase, the fraction of the cell cycle occupied by the C period decreases, whereas the fraction occupied by the B period increases and the D period remains nearly constant ( Supplementary Fig. S6e ). In contrast to the canonical organization of the cell division cycle as discrete and non-overlapping B, C and D periods [25] ( Fig. 6a ), we find that the B period is unusually short or absent in single cells of M. smegmatis ( Supplementary Fig. S6a and Supplementary Table S1 ). Thus, in the majority of single cells, the D period of the cell division cycle in the mother cell overlaps with the C period of the division cycle in the next-generation daughter cells ( Fig. 6b ). In our experiments, initiation of DNA replication in the mother cell before cytokinesis cannot be attributed to multifork replication [26] , [27] , [28] because we never observe a new round of DNA replication to initiate until the previous round has finished. 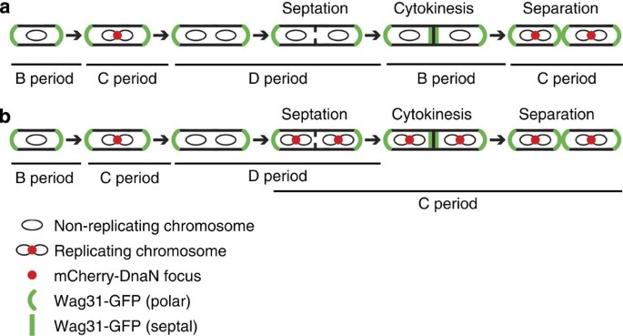Figure 6: Schematic of theM.smegmatiscell cycle. Schematic based on time-lapse microscopy experiments withM.smegmatisreporter strains expressing Wag31-GFP as a marker of cytokinesis and mCherry-DnaN as a marker of the DNA replisome. The division septum is visualized by staining cells with the fluorescent membrane dye FM4-64. (a) Canonical cell cycle organization comprising discrete B period (from cytokinesis to the initiation of chromosome replication), C period (from initiation to termination of chromosome replication) and D period (from termination of chromosome replication to cytokinesis). Chromosome replication occurs once per cell division cycle and initiation of chromosome replication does not occur until after cytokinesis of the mother cell. This pattern is exhibited by 22% (32/150) of cells. (b) Non-canonical cell cycle organization with overlapping D and C periods and no intervening B period. Chromosome replication occurs only once per cell division cycle, but chromosome replication initiates prior to cytokinesis of the mother cell. This pattern is exhibited by 78% (118/150) of cells. In a minority of cells (not depicted), a mixed pattern is observed in which one of the segregated chromosomes initiates replication prior to cytokinesis, whereas the other chromosome initiates replication after cytokinesis. Figure 6: Schematic of the M . smegmatis cell cycle. Schematic based on time-lapse microscopy experiments with M . smegmatis reporter strains expressing Wag31-GFP as a marker of cytokinesis and mCherry-DnaN as a marker of the DNA replisome. The division septum is visualized by staining cells with the fluorescent membrane dye FM4-64. ( a ) Canonical cell cycle organization comprising discrete B period (from cytokinesis to the initiation of chromosome replication), C period (from initiation to termination of chromosome replication) and D period (from termination of chromosome replication to cytokinesis). Chromosome replication occurs once per cell division cycle and initiation of chromosome replication does not occur until after cytokinesis of the mother cell. This pattern is exhibited by 22% (32/150) of cells. ( b ) Non-canonical cell cycle organization with overlapping D and C periods and no intervening B period. Chromosome replication occurs only once per cell division cycle, but chromosome replication initiates prior to cytokinesis of the mother cell. This pattern is exhibited by 78% (118/150) of cells. In a minority of cells (not depicted), a mixed pattern is observed in which one of the segregated chromosomes initiates replication prior to cytokinesis, whereas the other chromosome initiates replication after cytokinesis. Full size image Cell-size variation and size homoeostasis The origins and consequences of variation in the birth size, division size and interdivision time of single cells is a much-debated problem in cell biology [29] , [30] , [31] . At the single-cell level, we observe a strong scaling relationship between elongation rates and interdivision times, such that fast-growing individuals have shorter interdivision times than slow-growing individuals ( Fig. 5c ). These observations are inconsistent with a model in which the mycobacterial cell division cycle is governed by time [15] . On the other hand, the elongation lengths of single cells between birth and division ( L d – L b ) show only a weak positive correlation with the length at birth ( L b ) ( Fig. 7a ), and the length at division ( L d ) is positively correlated with L b ( Fig. 7b ). These observations are inconsistent with a ‘strict’ size-control mechanism that would trigger cell division once a critical cell size is achieved [16] . Nonetheless, our data suggest that some form of size control must be operational in mycobacteria because the interdivision time of single cells ( Fig. 7c ) and the fold-increase in cell size from birth to division ( L d )/( L b ) ( Fig. 7d ) are negatively correlated with L b . 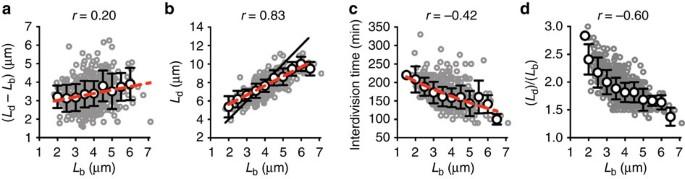Figure 7: Cell-size variation and size homoeostasis. (a-d) Time-lapse microscopy of bacteria expressing Wag31-GFP. Images recorded at 10-min intervals. This experiment was repeated three times with similar results. Graphs depict birth length (Lb) versus (a) elongation length from birth to next division (r=0.20), (b) length at division (r=0.83), (c) interdivision time (r=−0.42) and (d) fold-increase in length between birth and next division (r=−0.60). Grey circles represent single-cell values. Black circles represent mean values±s.d. for cells binned byLb. Dashed red line, data fitted to a linear function. In theLdversusLbplot, the black solid line represents theoretical fit of the data for cells that precisely double their length before dividing.rvalues, Pearson's correlation coefficient (n=520). Figure 7: Cell-size variation and size homoeostasis. ( a - d ) Time-lapse microscopy of bacteria expressing Wag31-GFP. Images recorded at 10-min intervals. This experiment was repeated three times with similar results. Graphs depict birth length ( L b ) versus ( a ) elongation length from birth to next division ( r =0.20), ( b ) length at division ( r =0.83), ( c ) interdivision time ( r =−0.42) and ( d ) fold-increase in length between birth and next division ( r =−0.60). Grey circles represent single-cell values. Black circles represent mean values±s.d. for cells binned by L b . Dashed red line, data fitted to a linear function. In the L d versus L b plot, the black solid line represents theoretical fit of the data for cells that precisely double their length before dividing. r values, Pearson's correlation coefficient ( n =520). Full size image Rod-shaped bacterial cells possess a new cell pole, arising from the most recent division event, and an old cell pole, arising from some previous division event. Recently, it was reported that mycobacteria grow in an unusual unipolar manner such that elongation occurs exclusively from the old cell pole [15] . Our observations are inconsistent with unipolar growth because we find that the old and new poles of individual cells elongate at the same velocity following cell separation ( Fig. 3b,c ). We also find that the fluorescence intensity of septal Wag31-GFP gradually increases during the period between its initial appearance at the nascent division septum (which coincides with cytokinesis) and the physical separation of the newborn sibling cells ( Fig. 2b ). This pattern of accumulation might reflect ongoing recruitment of the peptidoglycan synthesis/modification machinery required to initiate elongation of the new cell poles following cell separation [19] . These observations suggest that physical separation of sibling cells might be required for the initiation of growth from the new cell poles, consistent with the observation that mycobacteria elongate by inserting new cell-wall material exclusively at the cell poles [10] . In E. coli , cytokinesis and separation of daughter cells are nearly contemporaneous [32] . In mycobacteria, the lengthy delay between these events ( Fig. 2d ) underscores the importance of using validated markers, such as Wag31-GFP, to determine the timing of cytokinesis in single-cell experiments. Several recent studies, including this one, have demonstrated that rod-shaped mycobacteria usually divide asymmetrically, giving rise to sibling cells of unequal sizes [15] , [16] , [17] . In most cell divisions, displacement of the septum towards the newly formed cell pole causes the old-pole sibling to be larger than the new-pole sibling at birth. Although the mechanism responsible for asymmetric division is unclear, we can envisage two alternative scenarios, which are not mutually exclusive. In the first scenario, the nascent septum is initially localized accurately at midcell; however, preferential elongation of the old cell pole during the period from septum positioning to cytokinesis results in unequally sized sibling cells [15] , [16] . This explanation seems inconsistent with our observation that both cell poles elongate with the same velocity following cell separation ( Fig. 3c,d ). Moreover, during the early stages of septum formation, visualized as an FM4-64-stained membrane invagination, we find that the septum is already placed asymmetrically. Similarly, it has been shown that initial positioning of the FtsZ ring, one of the earliest recognizable events in division-site selection, is also asymmetric [12] . These observations tend to support a second scenario in which asymmetric division is because of initially skewed positioning of the division septum towards the new cell pole rather than at midcell. However, we cannot exclude the possibility that the position of the septum is already specified by other factors, as yet unknown, prior to the appearance of the FtsZ ring or FM4-64-stained invagination. If the future division site is specified during the period between cytokinesis of the mother cell and physical separation of the daughter cells ( Figs 2d and 3c ), exclusive growth of the old pole during this post-cytokinesis/pre-separation period could result in displacement of the septum away from the midcell position. In either scenario, the mechanism responsible for division-site selection is unknown. Although proteins equivalent to the well-characterized minicell and nucleoid occlusion systems are apparently absent in mycobacteria [33] , new factors such as the chromosome-partitioning protein ParA have been postulated to have a role in septum positioning [34] . In future experiments, it will be informative to employ reporter strains expressing multiple fluorescently tagged division proteins in order to determine the relative timing of appearance of these markers at the future site of cell division. Compared with better-characterized model organisms, there have been few studies on the organization of the DNA replication and cell division cycles in mycobacteria, particularly at the single-cell level. The real-time single-cell analysis presented here reveals some unusual features of the mycobacterial cell cycle that could not have been uncovered by population-based measurements. For example, a previous population-based study reported that the average duration of the C period in M. smegmatis is ∼ 110 min in batch cultures growing with a population doubling time of ∼ 180 min [35] . The fact that the average C period duration is less than the average interdivision time suggests a canonical organization of the mycobacterial cell cycle with discrete B, C and D periods [25] . Nonetheless, we find that in the majority of cell cycles, the B period is absent because chromosome replication initiates in the mother cell prior to cytokinesis and terminates in the daughter cells following cytokinesis ( Fig. 6b ). This observation is surprising because M. smegmatis apparently does not undergo multifork replication—that is, in M. smegmatis a new round of chromosome replication does not initiate until the previous round of replication has terminated. In other organisms that eschew multifork replication, such as C. crescentus , complex mechanisms have evolved to ensure that chromosome replication does not initiate before cell division has been completed [1] , [2] . In our experiments, single cells display marked cell-to-cell heterogeneity in their growth rates and interdivision times, which is accompanied by expansion or contraction of the C period and, to a lesser extent, of the B and D periods. Of note, the B period, which is absent in the majority of the cells, can occupy up to 20% of the cell cycle in the most slowly growing individuals. At present, it is unclear why the duration of the C period scales with the growth rates and interdivision times of individual cells. We speculate that the pools of precursors required for DNA synthesis might be kinetically limiting in slowly growing cells. Trial of this hypothesis awaits the development of methods for real-time single-cell measurements of the relevant metabolites in living mycobacteria. A long-standing debate in cell biology revolves around the question whether individual cells increase their size in a linear (size-independent) or exponential (size-dependent) manner [3] , [4] . Recent studies suggest that single cells of E. coli and B. subtilis grow in a size-dependent and approximately exponential manner [5] , [7] . Although the growth of mycobacteria by tip elongation might suggest that individual cells should increase their size in a linear manner [14] , our data reveal that mycobacteria elongate in a size-dependent manner. These results suggest that the size of the growth zone, which increases continuously in cells that grow by insertion of new material into the cell sidewalls (such as E. coli and B. subtilis ) but not in organisms that grow by insertion of new material into the cell tips (such as mycobacteria), is probably not rate-limiting for cell growth. In principle, size-dependent growth could be sufficient to explain why larger old-pole cells elongate at faster velocities than their smaller new-pole siblings, without invoking any additional mechanisms to account for this difference. Consistent with this interpretation, we find that the elongation velocity of individual cells is linked to cell size at birth rather than pole age per se ( Fig. 3g,h ). Thus, comparing new-pole and old-pole cells that are born at similar sizes, we find no significant difference in their elongation velocities. We also find no significant difference in the antibiotic sensitivity of new-pole versus old-pole cells, in contrast to a recent report that old-pole cells are more sensitive than new-pole cells to antibiotics that target cell-wall biogenesis [15] . At present, we cannot explain this discrepancy, although differences in the culture conditions and microfluidic devices used in the previous and present studies could conceivably affect cellular physiology and antibiotic sensitivity. All cells must coordinate the continuous process of cell growth (increase in biomass) with the discontinuous processes of chromosome replication/segregation and cell division/separation in order to maintain constant frequency distributions of ploidy and cell size. How this balance is achieved and maintained remains one of the major unresolved questions in microbial cell biology. The data presented here support neither a model in which the mycobacterial cell division cycle is governed by time (which implies that cells divide at defined time intervals, irrespective of their size) [15] nor a ‘strict’ size-control mechanism (which implies that cells divide once they attain a specific critical size) [16] . An alternative mechanism linking cell size and cell division is suggested by the observed correlation between cell size at birth and the fold-increase in cell size between birth and next division ( Fig. 7d ). These relationships imply that cells that are smaller than average at birth more than double their size before dividing, whereas cells that are larger than average at birth divide before doubling their size. These observations suggest that a ‘sloppy’ size-control mechanism [36] , [37] might be responsible for maintaining a stable frequency distribution of cell sizes in mycobacteria. According to this model, cells must achieve a certain minimal size before they are licensed to divide, and division is then a random process with size-dependent probability. Indeed, size-dependent growth of single cells implies that some mechanism of cell-size homoeostasis must exist; otherwise, the cell-to-cell size variation within a population would increase continuously from generation to generation, without limit [36] , [37] . Bacterial strains and culture conditions M. smegmatis mc 2 155 (wild type) and derivative strains were grown in Middlebrook 7H9 liquid medium (Difco) supplemented with 0.5% albumin, 0.2% glucose, 0.085% NaCl, 0.5% glycerol and 0.05% Tween-80. Cultures were grown at 37 °C to mid-log phase (optical density (OD 600 ) ∼ 0.5). Aliquots were stored in 15% glycerol at −80 °C and thawed at room temperature before use; individual aliquots were used once and discarded. Plasmids and oligonucleotides All plasmids and oligonucleotides used in this study are listed in Supplementary Table S2 . mCherry-DnaN reporter A reporter strain expressing a mCherry-DnaN fusion protein was constructed for single-cell imaging of the bacterial replisome. Regions of the M. smegmatis genome ∼ 600 bp upstream and downstream of the dnaN translational start codon were PCR-amplified from wild-type M. smegmatis genomic DNA using the oligonucleotide pairs dnaN_UPF/dnaN_UPR and dnaN_DnF/dnaN_dnR, respectively. PCR products were ligated into pCR2.1-TOPO (Invitrogen) and confirmed using DNA sequencing. Upstream and downstream fragments were released from pCR2.1-TOPO by restriction with Pac I/ Ssp I and Ssp I/ Xho I, respectively, and inserted between the Pac I and Xho I restriction sites in the allelic exchange suicide vector pJG1100, which contains the aph (kanamycin resistance), hyg (hygromycin resistance) and sacB (sucrose sensitivity) markers, to generate plasmid pIS147. The mCherry open reading frame (ORF) was PCR-amplified from pBS34 using the oligonucleotide pair m-ch_dnaN_F and m-ch_dnaN_R, digested with Eco RV, and inserted into Ssp I-digested pIS147 to generate plasmid pIS225. Correct orientation of mCherry was confirmed using restriction analysis and sequencing. Wag31-GFP and Wag31-mCherry reporters Reporter strains expressing a Wag31-GFP or Wag31-mCherry fusion protein were constructed for single-cell imaging of the bacterial cell division septum. The wag31 ORF (minus start and stop codons) was PCR-amplified from wild-type M. smegmatis genomic DNA using primers Wag31_F and Wag31_R, ligated into pCR2.1-TOPO (Invitrogen), and confirmed using DNA sequencing. The wag31 fragment was released from pCR2.1-TOPO by restriction with Nhe I and ligated into Nhe I-digested plasmid pND235 upstream of the gfp ORF to generate pIS216, or ligated into Nhe I-digested pIS232 upstream of the mCherry ORF to generate pIS236. Correct orientation of wag31 was confirmed using restriction analysis and DNA sequencing. The wag31::gfp (pIS216) or wag31::mCherry (pIS236) fragment was prepared for subcloning by restriction with Eco RI and end blunting with Klenow polymerase, followed by restriction with Pac I and end blunting with T4 DNA polymerase. The blunt-end fragments were ligated into Xmn I-digested plasmid pMV361 (a single-copy attB -integrating vector) downstream of the hsp60 transcriptional promoter to generate plasmids pIS220 ( wag31::gfp ) and pIS233 ( wag31::mCherry ). To generate plasmid pIS226, which was used in FLiP experiments, a fragment containing the DsRed ORF downstream of a strong constitutive promoter was released by restriction of plasmid pND239 with Ssp I and Cla I and ligated into Pvu II/ Cla I-digested pIS220. M. smegmatis fluorescent reporter strains An M. smegmatis strain expressing a mCherry-DnaN fusion protein was constructed using a method for two-step homologous recombination [38] , [39] with plasmid pIS225, which was inserted into the chromosome of wild-type M. smegmatis by electroporation with 1–2 μg of purified plasmid DNA. Electrocompetent M. smegmatis was prepared by growing bacteria to mid-log phase (OD 600 ∼ 0.5) in 7H9 liquid medium, washing three times with 10% glycerol and resuspending the washed cell pellet in 10% glycerol at 1/10th the original culture volume. Electroporated cells were grown for 3–6 h in 7H9 medium and plated on LB solid medium containing 15 μg ml −1 kanamycin and 50 μg ml −1 hygromycin to select for recombinants. Kan R /Hyg R colonies were picked and subcultured in 7H9 medium without antibiotics to mid-log phase (OD 600 ∼ 0.5). Integration of the plasmids at the dnaN locus via the upstream and downstream regions of homology was confirmed using colony PCR with oligonucleotide pairs dnaN_seq_UPF/mch_DnF plus dnaN_seq_DnF/mch_UPR, respectively. Clones that contained pIS225 integrated at the dnaN locus were plated on LB solid medium containing 5% sucrose for counterselection of the pJG1100 vector. Sucrose-resistant clones were subcultured in 7H9 medium, and isolates in which the wild-type dnaN gene was replaced by the mCherry::dnaN fusion gene were identified by PCR amplification with plasmid pairs dnaN_seq_UPF/mch_DnF plus dnaN_seq_DnF/mch_UPR and dnaN_seq_UPF plus dnaN_seq_DnR. Reporter strains with pIS220 ( wag31::gfp ) or pIS235 ( wag31::mCherry ) integrated at the chromosomal attB site were constructed by electroporating wild-type or mCherry::dnaN strains of M. smegmatis with 1–2 μg of plasmid DNA and selecting transformants on LB solid medium containing 15 μg ml −1 kanamycin. A reporter strain with pIS226 ( DsRed ) integrated at the chromosomal attB site was constructed by electroporating wild-type M. smegmatis with 1–2 μg of plasmid DNA and selecting transformants on LB solid medium containing 15 μg ml −1 kanamycin. Time-lapse fluorescence microscopy Bacteria were grown to the mid-log phase (OD 600 ∼ 0.5) in 7H9 medium, collected by centrifugation (2,400 g , 5 min), concentrated 10-fold in fresh 7H9 medium (37 °C) and passed through a 5-μm pore size PVDF syringe filter (Millipore) to remove clumps. The de-clumped cell suspension was spread on a coverslip, covered with a semipermeable membrane and cultured in a custom-made PDMS-based microfluidic device with continuous flow of 7H9 medium at 37 °C, as described [17] . Bacteria growing within the microfluidic device were imaged with the help of time-lapse microscopy using a DeltaVision personalDV inverted fluorescence microscope (Applied Precision) equipped with a 100 ° oil immersion objective and an environmental chamber maintained at 37 °C. Bacteria were fed by continuous flow of 7H9 medium with or without addition of 0.2 μg ml −1 of the red-fluorescent membrane dye FM4-64 (Invitrogen) at a flow rate of 25 μl min −1 . Images were recorded every 10 min on phase-contrast and fluorescence channels (for GFP, excitation filter 490/20/, emission filter 528/38/; for mCherry, excitation filter 575/25, emission filter 632/60) using a CoolSnap HQ2 camera. Images were processed using Softworx software (Applied Precision). Cell length was measured as the sum of short linear segments tracking along the centreline of individual cells in order to accommodate irregularities in cell shape. Length at birth ( L b ) was defined as the distance between polar and septal Wag31-GFP markers at the time of first appearance of Wag31-GFP signal at the septal position. Length at division ( L d ) was defined as the distance between the two polar Wag31-GFP markers at the time of first appearance of Wag31-GFP signal at the septal position. Interdivision time ( I t ) was defined as the time between the appearance of septal Wag31-GFP at the time of birth and the next appearance of septal Wag31-GFP at the time of division. Elongation velocity averaged over the lifetime of the cell was defined as ( L d − L b )/ I t . Elongation rate averaged over the lifetime of the cell was defined as ( L d / L b )/ I t . Elongation rate averaged over a specific time interval was defined as ( L n / L i )/( t n − t i ), where L i is the initial cell length at time t i , and L n is the cell length at a later time t n . Antibiotic exposure M. smegmatis expressing Wag31-GFP was cultured in a microfluidic device with continuous flow of 7H9 medium (37 °C) for 15 h to establish clonal microcolonies. The flow medium was then switched to 7H9 medium containing 20 μg ml −1 meropenem (LKT Laboratories), 200 μg ml −1 D-cycloserine (Sigma), 50 μg ml −1 isoniazid (Sigma) or 60 μg ml −1 rifampicin (Sigma), and incubation was continued for another 8 h. The flow medium was then switched to the 7H9 medium without antibiotic for another 8 h to permit recovery and outgrowth of surviving cells, and survival was scored as the percentage of cells that resumed growth after antibiotic washout. Throughout the time course, cells were imaged on the phase-contrast and fluorescence channels at 10-min intervals. FLiP assays For FLiP experiments, bacteria harbouring plasmid pIS226 (expressing DsRed2 from the UV15A promoter) or pND235 (expressing GFP from the UV15A promoter) were grown in a microfluidic device for 12 h (37 °C) in 7H9 medium or 7H9 medium plus 0.2 μg ml −1 FM4-64, respectively. Bacteria were imaged on phase-contrast and fluorescence channels and then pulse-bleached with a 488-nm laser or 532-nm laser focused at one end of the cell for 50 ms and 10–50% laser intensity (radius of the spot was 0.5 μm). Immediately afterwards, fluorescence images of the bleached cells were taken every 2 s for 30 s. Images were acquired using the DeltaVision version 2.10 software. We refer to the end of the cell that received the laser pulse as the ‘proximal end’ and the other end of the cell as the ‘distal end’. Using the ‘edit polygon’ function of the DeltaVision version 2.10 software, we defined individual polygons to represent the following: background fluorescence, bleached area of the target cell, unbleached area of the target cell, entire area of the control cell (a cell in close proximity to the target cell) and entire microcolony. The mean background (extracellular) fluorescence value was measured at each time point and this value was subtracted from the measured intracellular values prior to data processing. Repeated fluorescence imaging resulted in gradual photobleaching of the entire microcolony. To compensate for this effect, we measured the fluorescence of the entire microcolony at each time point following the laser pulse. Data obtained from each time point were then multiplied by a correction factor calculated as the ratio of microcolony fluorescence immediately after the laser pulse divided by the microcolony fluorescence at the matched time point. The percent change in intensity was calculated for the area of the unbleached region (ΔId) of the target cell and for the entire area of the control cell (ΔIc) before and after the laser pulse and normalized to the percent change in intensity of the bleached region (ΔIb) of the target cell by applying the formula: (ΔId/ΔIb) ° 100 or (ΔIc /ΔIb) ° 100. In the same cell, the mean intensity of fluorescence of septal FM4-64 or septal Wag31-GFP protein was measured and subtracted by the background value, which was measured inside the same cell but in a region not including the septum. In the graphs in Fig. 2c and Supplementary Fig. S1e , we plotted the (ΔId/ΔIb) ° 100 or (ΔIc/ΔIb) ° 100 versus the mean intensity of fluorescence of the Wag31-GFP protein or FM4-64 at the septum position of the cell. To track the time-dependent change in septal FM4-64 and septal Wag31-GFP fluorescence intensity, we defined individual polygons circumscribing the cell septum position and measured the mean intensity of fluorescence within the polygon every 10 min. Cell-wall labelling Cell-wall labelling of M. smegmatis followed a protocol described previously [15] . Briefly, a strain of M. smegmatis expressing the Wag31-mCherry fluorescent fusion protein was grown in the 7H9 liquid medium (37 °C) to the mid-log phase (OD 600 ∼ 0.5), collected by centrifugation (2,500 g , 5 min), washed with phosphate-buffered saline containing 0.2% Tween-20 (PBST) and resuspended in PBST at 1/10th the original culture volume. Alexa Fluor 488 carboxylic acid succinimidyl ester (Invitrogen) was added to a final concentration of 0.05 mg ml −1 and the cell suspension was gently mixed. The stained cells were immediately collected by centrifugation (2,500 g , 5 min), washed in PBST, resuspended in fresh 7H9 medium and transferred to a custom-made microfluidic device [17] . The stained bacteria were fed by a continuous flow of 7H9 medium (37 °C) and imaged on the phase-contrast and fluorescence channels (for GFP, excitation filter 490/20/, emission filter 528/38/; for mCherry, excitation filter 575/25, emission filter 632/60) every 10 min. Statistical analysis Mann–Whitney test was used to compare the elongation of the old and new cell poles ( Fig. 3d and Supplementary Fig. S2c ) and to compare the elongation of ‘pole 1’ and ‘pole 2’ ( Supplementary Fig. S2b ). Student's unpaired t -test was used to compare the growth parameters of old-pole and new-pole cells ( Fig. 4a–c ; Supplementary Fig. S3a–d ) and to compare the growth parameters of cells with different pole ages ( Supplementary Fig. S4a–d ). Fisher’s exact test was used to compare the survival probabilities of old-pole and new-pole cells exposed to antibiotics ( Fig. 4d ). P -values <0.05 were considered significant. How to cite this article: Santi, I. et al. Single-cell dynamics of the chromosome replication and cell division cycles in mycobacteria. Nat. Commun. 4:2470 doi: 10.1038/ncomms3470 (2013).